Phosphotransferase-dependent accumulation of (p)ppGpp in response to glutamine deprivation inCaulobacter crescentus The alarmone (p)ppGpp is commonly used by bacteria to quickly respond to nutrient starvation. Although (p)ppGpp synthetases such as SpoT have been extensively studied, little is known about the molecular mechanisms stimulating alarmone synthesis upon starvation. Here, we describe an essential role of the nitrogen-related phosphotransferase system (PTS Ntr ) in controlling (p)ppGpp accumulation in Caulobacter crescentus . We show that cells sense nitrogen starvation by way of detecting glutamine deprivation using the first enzyme (EI Ntr ) of PTS Ntr . Decreasing intracellular glutamine concentration triggers phosphorylation of EI Ntr and its downstream components HPr and EIIA Ntr . Once phosphorylated, both HPr ∼ P and EIIA Ntr ∼ P stimulate (p)ppGpp accumulation by modulating SpoT activities. This burst of second messenger primarily impacts the non-replicative phase of the cell cycle by extending the G1 phase. This work highlights a new role for bacterial PTS systems in stimulating (p)ppGpp accumulation in response to metabolic cues and in controlling cell cycle progression and cell growth. To face the environmental changes, organisms have developed complex regulatory mechanisms that integrate stimuli and stresses. Once activated, these signalling pathways modulate essential cellular processes such as DNA replication, cell division or cell growth. For example, upon nutrient starvation, yeast cells access to a specific quiescent state that enhances stress resistance and survival [1] . Bacteria also select many strategies to survive in challenging environments. One of the most studied bacterial adaptations to harsh conditions is certainly the formation of endospores in Bacillus subtilis , which requires asymmetric cell division and differentiation of the prespore [2] . Other bacteria take advantage of their asymmetric cell division to adapt to starvation conditions. It is the case of the aquatic α-proteobacterium Caulobacter crescentus that divides asymmetrically to give birth to two different daughter cells: a chemotactically active motile swarmer cell and a sessile stalked cell. Whereas the stalked cell grows and reinitiates DNA replication immediately at birth to ultimately divide again, the newborn swarmer cell enters first into a pre-replicative (G1) phase ( Fig. 1a ). In nutrient-replete conditions, the G1/swarmer cell differentiates into a stalked cell (swarmer-to-stalked transition) and concomitantly initiates chromosome replication (G1-to-S transition) [3] . Upon nitrogen starvation, C. crescentus extends its swarmer phase to promote spreading and colonization of new environments [4] , [5] , [6] . Asymmetric cell division might be a strategy commonly used by α-proteobacteria to generate daughter cells with different cell fates [7] . 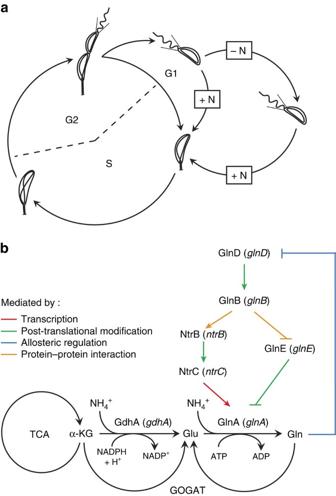Figure 1: TheC. crescentusswarmer cell lifetime is extended upon nitrogen starvation. (a) Asymmetric cell division ofC. crescentusgives birth to a non-replicative swarmer cell that goes through G1 phase before replicating and a replicative stalked cell that directly enters into S phase. Upon nitrogen starvation (−N), swarmer cells extend their G1 phase. (b) InE. coli, ammonium can be assimilated either by the NADP-dependent glutamate dehydrogenase (GdhA) to generate glutamate (Glu) from α-ketoglutarate (α-KG) or by the glutamine synthetase (GlnA) to produce glutamine (Gln) from Glu, this latter being recycled by the glutamate synthase (GOGAT). GlnA is regulated at different levels by the GlnD/GlnB/GlnE and NtrBC pathways, and GlnD senses intracellular pool of Gln. Figure 1: The C. crescentus swarmer cell lifetime is extended upon nitrogen starvation. ( a ) Asymmetric cell division of C. crescentus gives birth to a non-replicative swarmer cell that goes through G1 phase before replicating and a replicative stalked cell that directly enters into S phase. Upon nitrogen starvation (−N), swarmer cells extend their G1 phase. ( b ) In E. coli , ammonium can be assimilated either by the NADP-dependent glutamate dehydrogenase (GdhA) to generate glutamate (Glu) from α-ketoglutarate (α-KG) or by the glutamine synthetase (GlnA) to produce glutamine (Gln) from Glu, this latter being recycled by the glutamate synthase (GOGAT). GlnA is regulated at different levels by the GlnD/GlnB/GlnE and NtrBC pathways, and GlnD senses intracellular pool of Gln. Full size image Nutritional stresses are also known to be associated with the accumulation of an alarmone, the guanosine tetra- and penta-phosphate commonly called (p)ppGpp. Burst of intracellular (p)ppGpp alarmone allows cells to quickly adapt to a nutrient stress by affecting important cellular processes such as transcription, translation or DNA replication (reviewed in refs 8 and 9 ). For example, (p)ppGpp interferes with cell cycle steps by the direct binding of the alarmone to the DNA primase DnaG, which stops DNA replication in B. subtilis [10] . As a consequence of its pivotal role in stress adaptation, (p)ppGpp became crucial for virulence of several bacterial pathogens, long-term persistence, competence and biofilm formation [8] , [9] , [11] . In Escherichia coli , (p)ppGpp level is regulated by two proteins, RelA and SpoT [12] . RelA is a monofunctional (p)ppGpp synthetase stimulated by amino acids starvation, in contrast to SpoT, which is a bifunctional synthetase-hydrolase enzyme responding to a wide range of nutritional stresses such as carbon, phosphate or fatty acid starvation [9] . C. crescentus possesses a single RelA/SpoT homologue [12] that was named SpoT because of its bifunctional activity [13] , [14] . Previous studies showed that (p)ppGpp can modulate cell cycle progression in C. crescentus by delaying simultaneously the swarmer-to-stalked differentiation and the G1-to-S transition [13] , [15] , [16] . Nitrogen or carbon starvation was described to trigger accumulation of (p)ppGpp but the regulatory networks sensing these stresses and activating SpoT remain uncovered [13] , [14] . Furthermore, interacting partners of SpoT Cc are largely unknown even if SpoT Cc was shown to co-fractionate with the 70S ribosomal subunit [14] . Ammonium (NH 4 + ) is the preferred inorganic nitrogen source for most of living cells. There are only two reactions that efficiently assimilate NH 4 + ( Fig. 1b ). The first one is catalysed by the NADP-dependent assimilative glutamate dehydrogenase. The other one is mediated by the ATP-dependent glutamine synthetase (GlnA). There is no NADP-dependent glutamate dehydrogenase encoded in the genome of C. crescentus , suggesting that the assimilation of inorganic nitrogen is strictly dependent on the glutamine synthetase (GlnA) activity. In most bacteria, nitrogen metabolism is tightly regulated by a well-characterized pathway, which involves the universal nitrogen sensor GlnD ( Fig. 1b , reviewed in refs 17 and 18 ). When E. coli is grown in nitrogen-deplete (−N) conditions, the PII uridyltransferase GlnD catalyses the transfer of uridine monophosphate (UMP) groups to PII regulatory proteins, GlnB and GlnK. GlnK ∼ UMP no longer inhibits the ammonia channel AmtB, and GlnB ∼ UMP stimulates deadenylylation of GlnA by the adenylyltransferase GlnE, and thereby promotes glutamine synthetase activity ( Fig. 1b ). In nitrogen-replete (+N) conditions, GlnB inhibits the transcription of glnA , by stimulating dephosphorylation of the transcriptional activator NtrC, and promotes the addition of the adenine monophosphate groups by GlnE to GlnA, which slows down the glutamine synthetase activity ( Fig. 1b ). In this work, we unravel the regulatory network that stimulates (p)ppGpp accumulation in C. crescentus in response to nitrogen starvation. In particular, we uncover the essential role of the nitrogen-related phosphoenolpyruvate (PEP) phosphotransferase system (PTS Ntr ) in transducing glutamine deprivation signal to (p)ppGpp accumulation, which in turn controls the cell cycle progression. The cell cycle control described here constitutes a new PTS Ntr -dependent regulatory role, illustrating the diversity of the cellular processes regulated by PTS systems. Glutamine deprivation signals nitrogen starvation Previous studies showed that nitrogen starvation extends the swarmer cell lifetime in C. crescentus [4] , [5] , [6] . By following DNA content and cell cycle-regulated proteins (the flagellin and the stalked-associated protein StpX) in synchronous or asynchronous population of Caulobacter cells, we confirmed the specific extension of the G1/swarmer phase in response to nitrogen starvation ( Supplementary Fig. 1a–e ). By contrast, stalked cells can complete DNA replication once initiated, despite the absence of a nitrogen source ( Supplementary Fig. 1f ). To understand how nitrogen starvation affects the differentiation of G1/swarmer cells, we focused our work on proteins involved in nitrogen assimilation and metabolism. First, we created an in-frame deletion of the predicted gene coding for the general sensor for nitrogen availability, glnD (CCNA_00013). In contrast to wild-type cells, Δ glnD cells were unable to use ammonium as a nitrogen source. Indeed, the Δ glnD mutant did not grow and accumulated G1/swarmer cells when ammonium was used as the sole nitrogen source ( Supplementary Fig. 2a,b ). As expected, the G1 block and the growth were rescued in the presence of glutamine ( Supplementary Fig. 2 ). Indeed, as for glnD mutants in E. coli [19] , C. crescentus Δ glnD is auxotrophic for glutamine. Thus this result shows that G1/swarmer cells accumulation in Δ glnD is a consequence of its inability to use ammonium as a nitrogen source. Interestingly, the Δ glnD mutant strain cultivated in a complex peptone yeast extract (PYE) medium accumulated G1/swarmer cells ( Fig. 2c,d ). As a consequence, Δ glnD cells also exhibited (i) a slower growth than the wild-type strain and (ii) a bigger motility halo than the wild-type, despite the growth defect ( Fig. 2a,b ). Indeed, the overrepresentation of the G1/swarmer cells in a Δ glnD population increases the overall motility and the doubling time of the strain. Thus, our results indicate that G1/swarmer lifetime is extended in the absence of glnD ( Fig. 2a–d ). Again, addition of glutamine suppressed all these phenotypes ( Fig. 2d ), suggesting that defects of Δ glnD are a consequence of glutamine availability in the complex PYE medium. Indeed, PYE is mainly composed of yeast extract, in which glutamine is the less-abundant amino acid (≤0.2%, see the ‘Methods’ section). 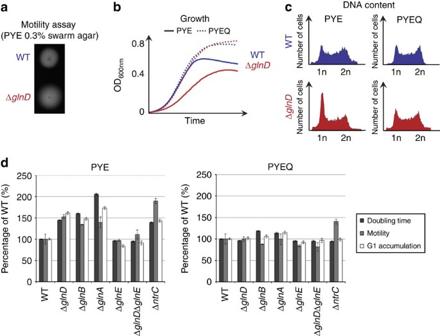Figure 2: TheC. crescentusG1/swarmer cell lifetime is dictated by intracellular glutamine concentration. (a–d) Extension of the G1/swarmer lifetime in a ΔglnDstrain can be compensated by addition of glutamine. Motility (a), growth (b) and DNA content (c) of wild-type (WT; RH50) and ΔglnD(RH577) grown in complex media without (PYE) or with glutamine (PYEQ) media. (d) G1/swarmer lifetime is extended in glutamine auxotrophic mutants. Doubling time, motility and G1 proportion were measured in WT (RH50), ΔglnD(RH577), ΔglnB(RH771), ΔglnA(RH772), ΔglnE(RH874), ΔglnDΔglnE(RH875) and ΔntrC(RH1458) grown in complex media without (PYE) or with glutamine (PYEQ), and normalized to the WT (100%). All these phenotypes can be rescued by addition of glutamine (PYEQ). Error bars=s.d.;n=3. Figure 2: The C. crescentus G1/swarmer cell lifetime is dictated by intracellular glutamine concentration. ( a – d ) Extension of the G1/swarmer lifetime in a Δ glnD strain can be compensated by addition of glutamine. Motility ( a ), growth ( b ) and DNA content ( c ) of wild-type (WT; RH50) and Δ glnD (RH577) grown in complex media without (PYE) or with glutamine (PYEQ) media. ( d ) G1/swarmer lifetime is extended in glutamine auxotrophic mutants. Doubling time, motility and G1 proportion were measured in WT (RH50), Δ glnD (RH577), Δ glnB (RH771), Δ glnA (RH772), Δ glnE (RH874), Δ glnD Δ glnE (RH875) and Δ ntrC (RH1458) grown in complex media without (PYE) or with glutamine (PYEQ), and normalized to the WT (100%). All these phenotypes can be rescued by addition of glutamine (PYEQ). Error bars=s.d. ; n =3. Full size image In E. coli , glutamine auxotrophy displayed by glnD mutant strains comes from the under-expression and lower activity of the glutamine synthetase GlnA. In the absence of GlnD, the PII protein GlnB is not uridylylated, and thereby constitutively stimulates (i) the dephosphorylation of transcriptional activator NtrC ∼ P by NtrB, which subsequently inhibits the NtrC ∼ P-dependent expression of glnA , and (ii) the adenylylation (+adenine monophosphate) of GlnA by the adenylytransferase GlnE, thereby inhibiting the glutamine synthetase activity ( Fig. 1b ). C. crescentus encodes three PII protein homologues ( glnB CCNA_02046, glnK CCNA_01400 and glnC CCNA_00555), one adenylytransferase homologue ( glnE CCNA_02839), three GlnA homologues ( glnA CCNA_02047, glnA 2 CCNA_03230 and glnA 3 CCNA_03240) and two NtrC homologues ( ntrC CCNA_01815, and ntrX CCNA_01817). Single in-frame deletions of each of these genes were created and tested for growth, motility and G1 accumulation in complex PYE medium. We found that only Δ glnB , Δ ntrC and Δ glnA recapitulated Δ glnD phenotypes, and that all these phenotypes could be suppressed by adding glutamine to the medium ( Fig. 2d ). However, it is noteworthy that the motility defect in Δ ntrC was not completely rescued by addition of glutamine, suggesting that NtrC also controls motility independently of G1/swarmer cells accumulation ( Fig. 2d ). Moreover, deleting glnE alleviated the Δ glnD defects, supporting the fact that inactivation (adenylylation) of GlnA by GlnE is the causative effect of the glutamine auxotrophy detected in Δ glnD cells ( Fig. 2d ). Unexpectedly, neither GlnA 2 nor GlnA 3 seems to participate in glutamine synthesis, at least in the conditions used here ( Supplementary Fig. 3a,b ). Finally, a catalytic mutant inactivating the glutamine synthetase activity of GlnA (GlnA R360A ) phenocopied Δ glnA in terms of glutamine auxotrophy, growth defect and G1 accumulation ( Supplementary Fig. 3c,d ), and all these defects can be suppressed by the addition of glutamine or complemented with a wild-type copy of glnA expressed in trans ( Supplementary Fig. 3d,e ). Altogether, these data support that (i) glutamine deprivation constitutes the signal for nitrogen starvation and that (ii) intracellular levels of glutamine drive the cell cycle progression of C. crescentus . Cell cycle response to nitrogen starvation requires (p)ppGpp To fish out key actors participating to the G1/swarmer extension in response to glutamine deprivation, we isolated spontaneous mutations that increase motility of the wild-type strain on PYE swarm agar plates supplemented with glutamine. Whole-genome sequencing of one candidate revealed a unique mutation (D81G) in the hydrolase domain of SpoT, the protein synthesizing (p)ppGpp ( Fig. 3a and Supplementary Fig. 4a ). It has been shown that mutations abolishing, at least partially, the hydrolase activity of SpoT without altering its synthetase activity, were all found in the hydrolase domain [20] . Interestingly, the conserved aspartate, corresponding to the D81 in C. crescentus SpoT, was found to be required for the hydrolase activity of SpoT in Streptococcus dysgalactiae [20] , which suggests that the D81G mutation may reduce hydrolase activity of SpoT in C. crescentus as well. The spoT D81G strain had a growth delay in PYE and accumulated G1/swarmer cells in exponential phase of growth ( Fig. 3b ; Supplementary Fig. 5a–c and Supplementary Movie 1 ), even when glutamine was added to the medium ( Supplementary Figs 5a–c and 6 ), confirming that the spoT D81G mutant is insensitive to glutamine. By contrast, in-frame deletion of spoT (Δ spoT ) displayed a motility defect on swarm agar and contained less G1/swarmer cells, in comparison with the wild-type ( Fig. 3b ; Supplementary Fig. 5b,c and Supplementary Movie 1 ). Most importantly, introducing Δ spoT in Δ glnD cells completely suppressed the accumulation of G1/swarmer cells ( Fig. 3b and Supplementary Fig. 5b,c ). This result highlights the role of (p)ppGpp produced by SpoT in response to glutamine deprivation to control the cell cycle. We thus checked the (p)ppGpp production in −N or +N conditions. In agreement with previous studies [14] , we found that (p)ppGpp concentration increases on glutamine deprivation, that is, in the wild-type strain grown without nitrogen source (−N) or in Δ glnD cultivated with (+N) or without (−N) NH 4 + ( Fig. 3c,d ; Supplementary Figs 1g and 5d ). As already mentioned in previous works [13] , [15] , we also observed a low amount of (p)ppGpp produced by wild-type cells in non-stressed conditions ( Fig. 3c and Supplementary Fig. 5d ). This (p)ppGpp steady-state level was slightly higher in the spoT D81G strain in +N conditions ( Fig. 3c and Supplementary Fig. 5d ), which would explain the phenotypes displayed by spoT D81G , that is, slower growth, bigger motility halo and G1 accumulation ( Fig. 3b ), even in the presence of glutamine ( Supplementary Figs 5a–c and 6 ). Nevertheless, spoT D81G cells accumulated similar levels of (p)ppGpp than wild-type cells upon nitrogen starvation (−N), suggesting that SpoT D81G is still sensitive to nitrogen starvation ( Fig. 3d ). In contrast, the disappearance of (p)ppGpp accumulated upon nitrogen starvation is slower in spoT D81G cells than in wild-type cells ( Supplementary Fig. 5e ). These results support that D81G mutation mainly affects the hydrolase activity of SpoT. It’s noteworthy that an artificial increase of (p)ppGpp levels in non-starved cells displayed similar phenotypes than spoT D81G in complex medium PYE [16] . The fact that, in non-stressed conditions, a strain producing more (p)ppGpp ( spoT D81G ) accumulated G1/swarmer cells, whereas a strain producing no (p)ppGpp at all (Δ spoT ) contained less G1/swarmer cells ( Fig. 3b,c ), suggest that (p)ppGpp steady-state level might determine the time spent by swarmer cells in G1 phase. Altogether, our findings indicate that glutamine deprivation increases (p)ppGpp level, which in turn, will extend the lifetime of G1/swarmer cells. 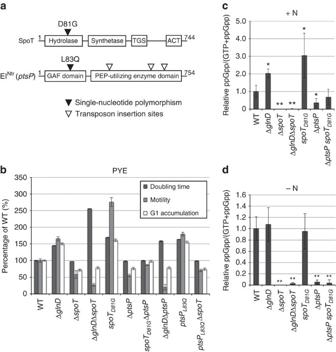Figure 3: SpoT and EINtrmodulate (p)ppGpp accumulation on nitrogen starvation. (a) Mutations isolated in SpoT and EINtrthat modulate G1/swarmer lifetime. Black arrowheads indicate the mutations (spoTD81GandptsPL83Q) that increase G1/swarmer lifetime. White arrowheads indicate the positions of 3himartransposon insertions in theptsPlocus out of the 16 that suppressedspoTD81Gphenotypes. The exact positions of the remaining 13 transposon insertions into theptsPlocus were not determined. (b) SpoT and EINtrcontrol G1/swarmer lifetime. Doubling time, motility and G1 proportion were measured in wild-type (WT; RH50), ΔglnD(RH577), ΔspoT(RH1755), ΔglnDΔspoT(RH1756),spoTD81G(RH1752), ΔptsP(RH1758), ΔptsP spoTD81G(RH1727) ΔglnDΔptsP(RH1940),ptsPL83Q(RH1748) and ΔspoT ptsPL83Q(RH1728) grown in complex media (PYE) and normalized to the WT (100%). Error bars=s.d.;n=3. (c,d) Glutamine auxotrophy leads to (p)ppGpp accumulation. Intracellular levels of (p)ppGpp detected by TLC after nucleotides extraction of WT (RH50), ΔglnD(RH577), ΔspoT(RH1755), ΔglnDΔspoT(RH1756),spoTD81G(RH1752), ΔptsP(RH1758) and ΔptsP spoTD81G(RH1727) grown (c) in +N or (d) −N conditions. Error bars=s.d.;n=3. Statistically significant differences by Student’st-test in comparison with the WT are indicated as *P<0.05% and **P<0.01% (n=3). Figure 3: SpoT and EI Ntr modulate (p)ppGpp accumulation on nitrogen starvation. ( a ) Mutations isolated in SpoT and EI Ntr that modulate G1/swarmer lifetime. Black arrowheads indicate the mutations ( spoT D81G and ptsP L83Q ) that increase G1/swarmer lifetime. White arrowheads indicate the positions of 3 himar transposon insertions in the ptsP locus out of the 16 that suppressed spoT D81G phenotypes. The exact positions of the remaining 13 transposon insertions into the ptsP locus were not determined. ( b ) SpoT and EI Ntr control G1/swarmer lifetime. Doubling time, motility and G1 proportion were measured in wild-type (WT; RH50), Δ glnD (RH577), Δ spoT (RH1755), Δ glnD Δ spoT (RH1756), spoT D81G (RH1752), Δ ptsP (RH1758), Δ ptsP spoT D81G (RH1727) Δ glnD Δ ptsP (RH1940), ptsP L83Q (RH1748) and Δ spoT ptsP L83Q (RH1728) grown in complex media (PYE) and normalized to the WT (100%). Error bars=s.d. ; n =3. ( c , d ) Glutamine auxotrophy leads to (p)ppGpp accumulation. Intracellular levels of (p)ppGpp detected by TLC after nucleotides extraction of WT (RH50), Δ glnD (RH577), Δ spoT (RH1755), Δ glnD Δ spoT (RH1756), spoT D81G (RH1752), Δ ptsP (RH1758) and Δ ptsP spoT D81G (RH1727) grown ( c ) in +N or ( d ) −N conditions. Error bars=s.d. ; n =3. Statistically significant differences by Student’s t -test in comparison with the WT are indicated as * P <0.05% and ** P <0.01% ( n =3). Full size image PTS Ntr promotes (p)ppGpp accumulation on nitrogen starvation To identify factors that participate to the activation of SpoT in response to nitrogen starvation, we selected for transposon insertions that improve growth of spoT D81G cells on complex medium (PYE). Indeed, the accumulation of (p)ppGpp in spoT D81G cells decreases the growth rate on PYE medium ( Fig. 3b and Supplementary Fig. 5a ). We identified multiple transposon insertions (34 out of 50 clones) into spoT D81G itself. The remaining 16 clones harboured a transposon insertion into the ptsP gene ( CCNA_00892 ), coding for a nitrogen-related PEP-phosphotransferase (PTS) protein homologue, called PtsP or EI Ntr in Enterobacteria ( Fig. 3a ). Canonical PTS systems are composed of several components that form a phosphorylation cascade initiated by autophosphorylation of the first protein called EI, using PEP as phosphoryl donor (reviewed in ref. 21 ). The phosphoryl group is then transferred from EI ∼ P to HPr and then to EIIA proteins. When the PTS system is used to take up sugars, the phosphoryl group is ultimately transferred from EIIA ∼ P to transported carbohydrates by using specific permeases (EIIB and EIIC components). In many other cases, PTS systems are dedicated to regulatory functions implying that PTS components (EI, HPr or EIIA) phosphorylate or interact with regulatory target proteins [21] . Nitrogen-related PTS (PTS Ntr ) systems are so far considered as unusual PTS systems that respond to nitrogen availability, but their regulatory roles in bacterial physiology remain poorly understood (reviewed in ref. 21 ). An in-frame deletion of ptsP in the parental spoT D81G strain suppressed the spoT D81G phenotypes, confirming the genetic interaction between ptsP and spoT D81G ( Fig. 3b ). In addition, Δ ptsP phenocopied Δ spoT in terms of motility, G1/swarmer cells accumulation ( Fig. 3b ; Supplementary Figs 5a–c and 7a–c ), and capability to suppress G1/swarmers cells accumulation of Δ glnD cells (compare Δ glnD Δ ptsP to Δ glnD Δ spoT in Fig. 3b ; Supplementary Figs 5a–c and 7a–c ). Interestingly, we isolated another candidate than spoT D81G in the gain-of-motility screen, which harboured a mutation (L83Q) in the GAF domain of EI Ntr ( ptsP L83Q ; Fig. 3a ). As ptsP L83Q phenocopies spoT D81G ( Fig. 3b ; Supplementary Figs 5a–c and 7a–c ), Δ ptsP suppresses spoT D81G defects and Δ spoT suppresses ptsP L83Q defects ( Fig. 3b ), we wondered whether ptsP (EI Ntr ) is upstream or downstream of spoT . To test that, we measured the (p)ppGpp levels in a spoT D81G Δ ptsP background. As shown in Fig. 3d , no (p)ppGpp accumulation was detected in spoT D81G Δ ptsP cells starved for nitrogen (−N). However, spoT D81G Δ ptsP cells still produced a low amount of (p)ppGpp, whether a nitrogen source was added to the medium or not ( Fig. 3c ). This constitutive low levels of (p)ppGpp produced by spoT D81G Δ ptsP cells is very close to the (p)ppGpp level detected in non-starved wild-type cells ( Fig. 3c ). Interestingly, there is a systematic correlation between the amount of (p)ppGpp produced by the cells and the time spent by these cells in G1 phase. Indeed, Δ spoT or Δ ptsP swarmer cells do not produce detectable levels of (p)ppGpp ( Fig. 3c ) and have shortened G1 phase ( Fig. 3b ), whereas spoT D81G Δ ptsP and wild-type cells have similar levels of (p)ppGpp and G1 lifetime ( Fig. 3b,c ). Altogether, these results support the role played by (p)ppGpp in determining the G1 lifetime, and show that EI Ntr regulates (p)ppGpp levels by controlling SpoT. Glutamine inhibits EI Ntr autophosphorylation To understand how glutamine deprivation is transduced to SpoT, we first looked at the autophosphorylation level of EI Ntr . Indeed, as described above, accumulation of G1/swarmer cells ( Fig. 3b ) observed in a ptsP L83Q background, are not compensated by supplying an exogenous source of glutamine ( Supplementary Fig. 6 ). Moreover, it has been recently shown, in the closely related α-proteobacterium Sinorhizobium meliloti , that binding of glutamine to the conserved N-terminal GAF domain of EI Ntr inhibits its autophosphorylation [22] . To check whether the phosphorylation of EI Ntr is also sensitive to glutamine in C. crescentus , we performed in vitro autophosphorylation assays with a purified fraction containing EI Ntr using [ 32 P]PEP as a phosphoryl donor, in the presence or absence of glutamine. We found that autophosphorylation of EI Ntr was strongly reduced by glutamine ( Fig. 4a and Supplementary Fig. 8a ). In contrast, autophosphorylation of the EI Ntr L83Q mutant form was not modulated by the presence of glutamine ( Fig. 4a ), suggesting that the mutation L83Q prevents glutamine binding to the highly conserved region of the EI Ntr GAF domain ( Supplementary Fig. 4b ). 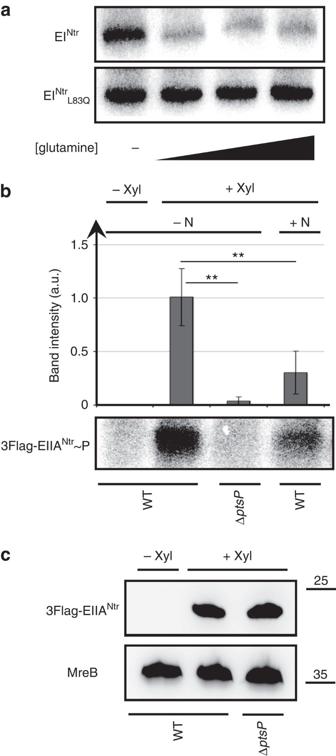Figure 4: Glutamine inhibits PTSNtrphosphorylation. (a) Glutamine inhibits autophosphorylation of EINtrbut not EINtrL83Q. Autophosphorylation assays of EINtrand EINtrL83Qusing [32P]PEP as a phosphoryl donor in the absence or presence of increasing concentration of glutamine (0, 2, 5, 10 mM). The full autoradiography is available inSupplementary Fig. 8a. (b) The EINtr-dependent phosphorylation of EIIANtris enhanced upon nitrogen starvation.In vivophosphorylation assays of EIIANtrin −N or +N conditions supplemented with (+Xyl) or without (−Xyl) xylose in wild-type (WT) or ΔptsPcells expressing3FLAG-ptsNfrom PxylXpromoter. Error bars=s.d.;n=3. Statistically significant differences by Student’st-test are indicated as **P<0.01% (n=3). The full autoradiography is available inSupplementary Fig. 8b. (c) Immunoblotting of protein samples extracted from WT and ΔptsPcells expressing3FLAG-ptsNfrom PxylXpromoter, incubated 3 h in M5GG supplemented with (+Xyl) or without (−Xyl) xylose. MreB was detected in all conditions, while 3FLAG-EIIANtrwas detected only in the presence of xylose. The full blot is available inSupplementary Fig. 8c. Figure 4: Glutamine inhibits PTS Ntr phosphorylation. ( a ) Glutamine inhibits autophosphorylation of EI Ntr but not EI Ntr L83Q . Autophosphorylation assays of EI Ntr and EI Ntr L83Q using [ 32 P]PEP as a phosphoryl donor in the absence or presence of increasing concentration of glutamine (0, 2, 5, 10 mM). The full autoradiography is available in Supplementary Fig. 8a . ( b ) The EI Ntr -dependent phosphorylation of EIIA Ntr is enhanced upon nitrogen starvation. In vivo phosphorylation assays of EIIA Ntr in −N or +N conditions supplemented with (+Xyl) or without (−Xyl) xylose in wild-type (WT) or Δ ptsP cells expressing 3FLAG-ptsN from P xylX promoter. Error bars=s.d. ; n =3. Statistically significant differences by Student’s t -test are indicated as ** P <0.01% ( n =3). The full autoradiography is available in Supplementary Fig. 8b . ( c ) Immunoblotting of protein samples extracted from WT and Δ ptsP cells expressing 3FLAG-ptsN from P xylX promoter, incubated 3 h in M5GG supplemented with (+Xyl) or without (−Xyl) xylose. MreB was detected in all conditions, while 3FLAG-EIIA Ntr was detected only in the presence of xylose. The full blot is available in Supplementary Fig. 8c . Full size image Phosphorylated PTS Ntr proteins trigger (p)ppGpp accumulation To unravel how EI Ntr controls SpoT activity, we first searched for components that could participate to PTS Ntr phosphorelay ( Fig. 5a ). Besides ptsP (EI Ntr ), we found a unique HPr homologue ( ptsH , CCNA_00241 ) and another nitrogen-related PTS Ntr component, EIIA Ntr ( ptsN , CCNA_03710 ). We created single in-frame deletions of the two genes (Δ ptsH and Δ ptsN ) and found that the proportion of G1/swarmer cells in Δ ptsH (without HPr) or Δ ptsN (without EIIA Ntr ) strain was reduced in comparison with the wild-type strain in complex medium ( Fig. 5b ), a phenotype already described for Δ ptsP (without EI Ntr ) and for Δ spoT ( Fig. 5b ). Interestingly, strains expressing a non-phosphorylatable version of EIIA Ntr (EIIA Ntr H66A ) accumulated G1 cells as much as the loss-of-function mutant (Δ ptsN ), that is, less than the wild-type strain ( Fig. 5b ), suggesting that the PTS Ntr pathway is slightly phosphorylated in complex medium PYE and that the last component of the PTS Ntr phosphorelay, EIIA Ntr , controls SpoT activity. 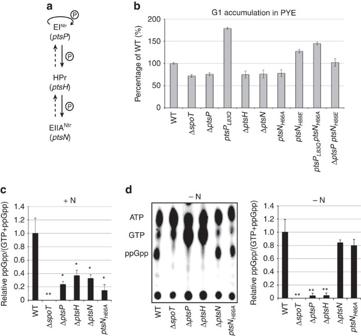Figure 5: PTSNtrmodulates (p)ppGpp accumulation. (a) Schematic representation of the PTSNtrpathway inC. crescentus. (b) The PTSNtrcomponents EINtr, HPr and EIIANtrcontrol G1/swarmer lifetime. G1 proportion was measured in wild-type (WT; RH50), ΔspoT(RH1755), ΔptsP(RH1758),ptsPL83Q(RH1748), ΔptsH(RH1621), ΔptsN(RH1819),ptsNH66A(RH2019),ptsNH66E(RH2017),ptsPL83QptsNH66A(RH2018), ΔptsP ptsNH66E(RH2016) grown in complex media (PYE) and normalized to the WT (100%). Error bars=s.d.;n=3. (c,d) (p)ppGpp accumulation is modulated by PTSNtr. Intracellular levels of (p)ppGpp detected by TLC after nucleotides extraction of WT (RH50), ΔspoT(RH1755), ΔptsP(RH1758), ΔptsH(RH1621), ΔptsN(RH1819) andptsNH66A(RH2019) grown (c) in +N or (d) −N conditions. Error bars=s.d.;n=3. Statistically significant differences by Student’st-test in comparison with the WT are indicated as *P<0.05% and **P<0.01% (n=3). Figure 5: PTS Ntr modulates (p)ppGpp accumulation. ( a ) Schematic representation of the PTS Ntr pathway in C. crescentus . ( b ) The PTS Ntr components EI Ntr , HPr and EIIA Ntr control G1/swarmer lifetime. G1 proportion was measured in wild-type (WT; RH50), Δ spoT (RH1755), Δ ptsP (RH1758), ptsP L83Q (RH1748), Δ ptsH (RH1621), Δ ptsN (RH1819), ptsN H66A (RH2019), ptsN H66E (RH2017), ptsP L83Q ptsN H66A (RH2018), Δ ptsP ptsN H66E (RH2016) grown in complex media (PYE) and normalized to the WT (100%). Error bars=s.d. ; n =3. ( c , d ) (p)ppGpp accumulation is modulated by PTS Ntr . Intracellular levels of (p)ppGpp detected by TLC after nucleotides extraction of WT (RH50), Δ spoT (RH1755), Δ ptsP (RH1758), Δ ptsH (RH1621), Δ ptsN (RH1819) and ptsN H66A (RH2019) grown ( c ) in +N or ( d ) −N conditions. Error bars=s.d. ; n =3. Statistically significant differences by Student’s t -test in comparison with the WT are indicated as * P <0.05% and ** P <0.01% ( n =3). Full size image To validate the conservation of PTS Ntr phosphorelay and the inhibitory effect of glutamine on this cascade, we checked the phosphorylation level of EIIA Ntr in +N or −N conditions. To this purpose, we performed in vivo phosphorylation assays on WT and Δ ptsP (without EI Ntr ) strains expressing a xylose-inducible tagged version of EIIA Ntr (P xylX::3FLAG-ptsN ; Fig. 4b,c and Supplementary Fig. 8b,c ). In agreement with our previous data, we found that the phosphorylation of EIIA Ntr is enhanced in the absence of nitrogen sources (−N) in comparison with the +N conditions ( Fig. 4b,c and Supplementary Fig. 8b,c ). In addition, we showed that EI Ntr is required in vivo for EIIA Ntr phosphorylation, since phosphorylated EIIA Ntr was undetectable in Δ ptsP cells starved for nitrogen ( Fig. 4b,c and Supplementary Fig. 8b,c ). In addition, we measured the (p)ppGpp levels in the single PTS Ntr mutants first in +N conditions. Consistent with the G1 accumulation in PYE, we found that PTS Ntr mutant strains (Δ ptsP , Δ ptsH , Δ ptsN or ptsN H66A ) produced significantly lower amount of (p)ppGpp than the wild-type strain in the presence of a nitrogen source ( Fig. 5c ). Moreover, EIIA Ntr H66A partially abrogated the cell cycle and developmental defects of ptsP L83Q (EI Ntr L83Q ) supporting the fact that overphosphorylation of EIIA Ntr in ptsP L83Q cells is partially responsible for (p)ppGpp accumulation and subsequent G1-to-S transition delay ( Fig. 5b ). On the contrary, a strain expressing a phosphomimetic mutant of EIIA Ntr (EIIA Ntr H66E ) had increased proportion of G1 cells independently of the presence of EI Ntr ( Fig. 5b ). Altogether, these data suggest that the phosphorylated form of EIIA Ntr (EIIA Ntr ∼ P) controls SpoT activity. However, (p)ppGpp measurements in −N conditions showed that SpoT is also controlled in an EIIA Ntr ∼ P-independent way. Indeed, in contrast to cells devoid of EI Ntr (Δ ptsP ) or HPr (Δ ptsH ), which did not accumulate (p)ppGpp upon nitrogen starvation ( Fig. 5d ), the absence of EIIA Ntr ∼ P in Δ ptsN or ptsN H66A cells did not abolish (p)ppGpp accumulation upon nitrogen starvation ( Fig. 5d ), showing that SpoT is still sensitive to nitrogen availability in the absence of EIIA Ntr ∼ P. On the basis of these results, we propose a model in which HPr ∼ P controls the intracellular levels of (p)ppGpp by at least two ways, in an EIIA Ntr ∼ P-dependent way but also independently of EIIA Ntr ∼ P. Phosphorylated EIIA Ntr directly interacts with SpoT Since most of the regulatory functions of PTS components are mediated by protein–protein interactions, we checked whether HPr and EIIA Ntr were able to interact with SpoT by performing bacterial two-hybrid (BTH) assays. To this end, T18 or T25 domains of Bordetella pertussis adenylate cyclase [23] were fused to coding sequences of HPr ( ptsH and ptsH H18A ), EIIA Ntr ( ptsN , ptsN H66A and ptsN H66E ) and SpoT ( spoT and spoT D81G ). We found that both the wild-type EIIA Ntr ( ptsN ) and the phosphomimetic mutant of EIIA Ntr (EIIA Ntr H66E ) were able to interact with SpoT versions ( Fig. 6a,b and Supplementary Fig. 9a ), while the non-phosphorylatable mutant EIIA Ntr H66A was not ( Fig. 6a,b and Supplementary Fig. 9a ). Both T18-EIIA Ntr H66A and T25-EIIA Ntr H66A can, respectively, interact with T25-HPr and T18-HPr ( Fig. 6c and Supplementary Fig. 9a ), showing that EIIA Ntr H66A is functional in the BTH assays. Altogether, these findings suggest that EIIA Ntr is phosphorylated in vivo in E. coli . Indeed, there are two PTS systems in E. coli , a canonical one composed of EI ( ptsI ), HPr ( ptsH ) and EIIA ( ptsM ), as well as a nitrogen-related one composed of EI Ntr ( ptsP ), NPr ( npr ) and EIIA Ntr ( ptsN ), and both pathways can cross-talk to some extent [24] ( Supplementary Fig. 9b ). To test whether Caulobacter EIIA Ntr is phosphorylated in vivo in E. coli , strains deleted for npr (NPr) or for both ptsP (EI Ntr ) and ptsI (EI) genes were created. As illustrated on Fig. 6a and Supplementary Fig. 9c , the interaction between EIIA Ntr and SpoT was abolished in the Δ npr strain while EIIA Ntr H66E retained the ability to interact with SpoT. Likewise, no more β-galactosidase activity was detected in a Δ ptsP Δ ptsI background (without E. coli EI proteins) expressing T25-SpoT and T18-EIIA Ntr , while the interaction between SpoT and EIIA Ntr H66E remained unchanged in this background ( Fig. 6b ). Finally, the expression of Caulobacter ptsH (HPr) from the inducible pBAD promoter (pBAD33 -ptsH Cc ) in a Δ npr background restored the interaction between EIIA Ntr and SpoT only when arabinose was added to the medium ( Supplementary Fig. 9c ), indicating that Caulobacter HPr and EIIA Ntr proteins can be phosphorylated by E. coli PTS systems, and that only the phosphorylated form of EIIA Ntr interacts with SpoT. In contrast to EIIA Ntr , no interaction was detected between HPr (or HPr H18A ) and SpoT (or SpoT D81G ) on MacConkey maltose agar plates ( Supplementary Fig. 9d ). The fact that HPr interacts with EIIA Ntr H66A ( Fig. 6c and Supplementary Fig. 9a ) shows that HPr is functional in the BTH assays. 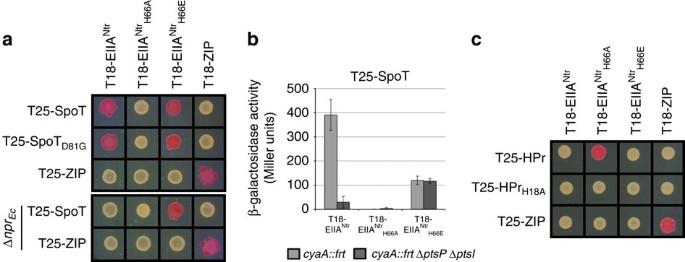Figure 6: The phosphorylated form of EIIANtrinteracts with SpoT in BTH assays. (a) In contrast to EIIANtrH66A, EIIANtr∼P and EIIANtrH66Edirectly interact with SpoT. MG1655cyaA::frt(RH785) or MG1655cyaA::frtΔnpr(RH2122) strains coexpressing T18- fused toptsN,ptsNH66A, ptsNH66EorZIPwith T25- fused tospoT,spoTD81GorZIPwere spotted on MacConkey agar base plates supplemented with 1% maltose and 1 mM IPTG. Plates were incubated for 3–4 days at 30 °C. The red colour indicates positive interactions. (b) The absence ofE. coliEI and EINtrproteins abolishes interaction between SpoT and EIIANtrbut not with EIIANtrH66E. β-galactosidase assays were performed on strains coexpressing T25-SpoT and T18-EIIANtr, T18-EIIANtrH66Aor T18-EIIANtrH66E, in the presence (MG1655cyaA::frt(RH785)) or absence (MG1655cyaA::frtΔptsPΔptsI(RH2124)) of EI and EINtrproteins. Error bars=s.d.;n=3. (c) In contrast to HPrH18A, HPr∼P directly interacts with EIIANtrH66A. MG1655cyaA::frt(RH785) strain coexpressing T18- fused toptsN,ptsNH66A, ptsNH66EorZIPwith T25- fused tohpr,hprH18AorZIPwere spotted on MacConkey agar base plates supplemented with 1% maltose and 1 mM IPTG. Plates were incubated for 3–4 days at 30 °C. The red colour indicates positive interactions. Figure 6: The phosphorylated form of EIIA Ntr interacts with SpoT in BTH assays. ( a ) In contrast to EIIA Ntr H66A , EIIA Ntr ∼ P and EIIA Ntr H66E directly interact with SpoT. MG1655 cyaA::frt (RH785) or MG1655 cyaA::frt Δ npr (RH2122) strains coexpressing T18- fused to ptsN , ptsN H66A , ptsN H66E or ZIP with T25- fused to spoT , spoT D81G or ZIP were spotted on MacConkey agar base plates supplemented with 1% maltose and 1 mM IPTG. Plates were incubated for 3–4 days at 30 °C. The red colour indicates positive interactions. ( b ) The absence of E. coli EI and EI Ntr proteins abolishes interaction between SpoT and EIIA Ntr but not with EIIA Ntr H66E . β-galactosidase assays were performed on strains coexpressing T25-SpoT and T18-EIIA Ntr , T18-EIIA Ntr H66A or T18-EIIA Ntr H66E , in the presence (MG1655 cyaA::frt (RH785)) or absence (MG1655 cyaA::frt Δ ptsP Δ ptsI (RH2124)) of EI and EI Ntr proteins. Error bars=s.d. ; n =3. ( c ) In contrast to HPr H18A , HPr ∼ P directly interacts with EIIA Ntr H66A . MG1655 cyaA::frt (RH785) strain coexpressing T18- fused to ptsN , ptsN H66A , ptsN H66E or ZIP with T25- fused to hpr , hpr H18A or ZIP were spotted on MacConkey agar base plates supplemented with 1% maltose and 1 mM IPTG. Plates were incubated for 3–4 days at 30 °C. The red colour indicates positive interactions. Full size image Altogether, these BTH data strongly suggest that (i) HPr and EIIA Ntr are both phosphorylated in E. coli and (ii) EIIA Ntr ∼ P is the only form of EIIA Ntr able to interact with SpoT, thereby supporting a model in which SpoT activity is controlled directly by EIIA Ntr ∼ P, and indirectly by HPr ∼ P ( Fig. 8 ). Figure 8: PTS Ntr -dependent accumulation of (p)ppGpp upon glutamine deprivation. 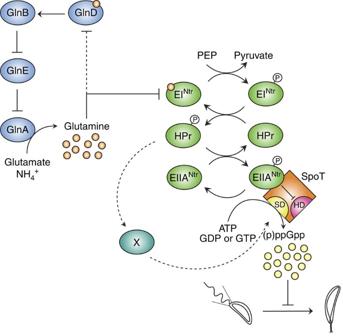Figure 8: PTSNtr-dependent accumulation of (p)ppGpp upon glutamine deprivation. The GlnD/GlnB/GlnE pathway (in blue) regulates glutamine homoeostasis by modulating GlnA (GS) activity. Intracellular glutamine inhibits EINtrautophosphorylation, limiting the (p)ppGpp production in +N conditions. Note that the GlnD activity is very likely also inhibited by intracellular glutamine. On nitrogen starvation, intracellular pool of glutamine drops, relieving inhibition of EINtrautophosphorylation and thereby increasing HPr and EIIANtrphosphorylation levels (in green). Once phosphorylated, EIIANtr∼P interacts with SpoT to inhibit its hydrolase activity (HD), whereas HPr∼P regulates indirectly SpoT synthetase activity (SD). This dual control of SpoT by HPr∼P and EIIANtr∼P leads to (p)ppGpp accumulation, which in turn delays the G1-to-S and swarmer-to-stalked cell transition. The GlnD/GlnB/GlnE pathway (in blue) regulates glutamine homoeostasis by modulating GlnA (GS) activity. Intracellular glutamine inhibits EI Ntr autophosphorylation, limiting the (p)ppGpp production in +N conditions. Note that the GlnD activity is very likely also inhibited by intracellular glutamine. On nitrogen starvation, intracellular pool of glutamine drops, relieving inhibition of EI Ntr autophosphorylation and thereby increasing HPr and EIIA Ntr phosphorylation levels (in green). Once phosphorylated, EIIA Ntr ∼ P interacts with SpoT to inhibit its hydrolase activity (HD), whereas HPr ∼ P regulates indirectly SpoT synthetase activity (SD). This dual control of SpoT by HPr ∼ P and EIIA Ntr ∼ P leads to (p)ppGpp accumulation, which in turn delays the G1-to-S and swarmer-to-stalked cell transition. Full size image Phosphorylated EIIA Ntr inhibits hydrolase activity of SpoT Interestingly, the deletion of ptsN (EIIA Ntr ) did not abolish the G1 accumulation of spoT D81G cells in contrast to Δ ptsP (EI Ntr ) or Δ ptsH (HPr; Fig. 7a ). The fact that SpoT D81G , which harbours a reduced hydrolase activity ( Supplementary Fig. 5e ), is insensitive to the presence of EIIA Ntr suggests that EIIA Ntr ∼ P might inhibit the hydrolase activity of SpoT rather than stimulating its synthetase activity. This could explain why Δ ptsN or ptsN H66A are still able to accumulate high levels of (p)ppGpp on nitrogen starvation, while Δ ptsP or Δ ptsH cannot ( Fig. 5d ). To validate our hypothesis, we engineered Caulobacter strains in which the only (p)ppGpp synthetase activity was supplied by the unrelated E. coli RelA protein, and we measured the endogenous hydrolase activity of SpoT in different genetic backgrounds. To this end, we first abolished the synthetase activity of SpoT in several backgrounds ( spoT D81G , ptsN H66A , ptsN H66E and Δ ptsP ), by replacing the tyrosine 323 of SpoT by an alanine (SpoT Y323A ; ref. 14 ). As expected, all these strains displayed a G1 accumulation similar to a Δ spoT strain in PYE complex medium ( Fig. 7c ). In a second time, we inserted a truncated version of E. coli RelA (p)ppGpp synthetase at the xylose locus, leading to an artificial (p)ppGpp accumulation in Caulobacter upon addition of xylose (P xylX::relA-FLAG ; ref. 16 ). Since the hydrolase domain of RelA is inactive, the only (p)ppGpp hydrolase activity in these strains was carried out by the Caulobacter SpoT protein, while the only (p)ppGpp synthetase activity was supported by the E. coli RelA protein. In the presence of xylose, both spoT D81G Y323A and ptsN H66E spoT Y323A displayed a growth defect and a G1 accumulation in comparison with the parental spoT Y323A strain ( Fig. 7b,c and Supplementary Fig. 10 ). On the contrary, neither ptsN H66A spoT Y323A nor Δ ptsP spoT Y323A strains had a growth delay or accumulated G1/swarmer cell upon xylose induction. These results strongly suggest that the phosphorylated form of EIIA Ntr ( ptsN ) specifically inhibits the hydrolase activity of SpoT. In support of this, we found that upon xylose induction ( Fig. 7d ), spoT Y323A P xylX::relA-FLAG cells accumulated (p)ppGpp in −N conditions (that is, when EIIA Ntr is highly phosphorylated; Fig. 4b ), but not in +N conditions (that is, when EIIA Ntr is less phosphorylated; Fig. 4b ). Furthermore, (p)ppGpp accumulated in spoT D81G Y323A P xylX::relA-FLAG cells even in +N conditions ( Fig. 7d ), supporting again that the D81G mutation abolishes the hydrolase activity of SpoT. Finally, (p)ppGpp became undetectable in spoT Y323A P xylX::relA-FLAG strains harbouring ptsN H66A or Δ ptsP allele ( Fig. 7d ), indicating that SpoT hydrolase activity is completely unlocked when EIIA Ntr is unphosphorylated. 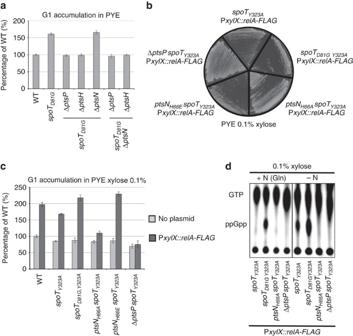Altogether, these findings demonstrate that EIIA Ntr ∼ P inhibits hydrolase activity of SpoT to modulate (p)ppGpp accumulation upon nitrogen availability. Figure 7: EIIANtr∼P inhibits the hydrolase activity of SpoT. (a)spoTD81Gis insensitive to the absence of EIIANtr. G1 proportion was measured in wild-type (WT; RH50),spoTD81G(RH1752),spoTD81GΔptsP(RH1727),spoTD81GΔptsH(RH2013),spoTD81GΔptsN(RH1999),spoTD81GΔptsNΔptsP(RH2014) andspoTD81GΔptsNΔptsH(RH2015) grown in complex media (PYE) and normalized to the WT (100%). Error bars=s.d.;n=3. (b) The hydrolase activity of SpoT is required for growth on an artificial exogenous production of (p)ppGpp. Growth ofspoTY323A, spoTD81G Y323A, ptsNH66AspoTY323A, ptsNH66EspoTY323Aand ΔptsP spoTY323Aexpressing a truncated version ofE. coli relAfrom the induciblexylXpromoter (PxylX::relA-FLAG) on PYE medium supplemented with 0.1% of xylose. (c) Reduction of SpoT hydrolase activity led to a G1 extension on an artificial exogenous production of (p)ppGpp. Flow cytometry analysis to determine DNA content in asynchronous population of WT,spoTY323A, spoTD81G Y323A, ptsNH66AspoTY323A, ptsNH66EspoTY323Aand ΔptsP spoTY323Awith (dark grey bars) or without (light grey bars) PxylX::relA-FLAGin PYE medium supplemented with 0.1% of xylose. The data were normalized to the WT without PxylX::relA-FLAG(100%). Error bars=s.d.;n=3. (d) The hydrolase activity of SpoT is required to degrade (p)ppGpp in +N condition. Intracellular levels of (p)ppGpp detected by TLC after nucleotides extraction ofspoTY323A, spoTD81G Y323A, ptsNH66AspoTY323Aand ΔptsP spoTY323Acontaining PxylX::relA-FLAGin +N or −N medium supplemented with 0.1% xylose. Figure 7: EIIA Ntr ∼ P inhibits the hydrolase activity of SpoT. ( a ) spoT D81G is insensitive to the absence of EIIA Ntr . G1 proportion was measured in wild-type (WT; RH50), spoT D81G (RH1752), spoT D81G Δ ptsP (RH1727), spoT D81G Δ ptsH (RH2013), spoT D81G Δ ptsN (RH1999), spoT D81G Δ ptsN Δ ptsP (RH2014) and spoT D81G Δ ptsN Δ ptsH (RH2015) grown in complex media (PYE) and normalized to the WT (100%). Error bars=s.d. ; n =3. ( b ) The hydrolase activity of SpoT is required for growth on an artificial exogenous production of (p)ppGpp. Growth of spoT Y323A , spoT D81G Y323A , ptsN H66A spoT Y323A , ptsN H66E spoT Y323A and Δ ptsP spoT Y323A expressing a truncated version of E. coli relA from the inducible xylX promoter (P xylX::relA-FLAG ) on PYE medium supplemented with 0.1% of xylose. ( c ) Reduction of SpoT hydrolase activity led to a G1 extension on an artificial exogenous production of (p)ppGpp. Flow cytometry analysis to determine DNA content in asynchronous population of WT, spoT Y323A , spoT D81G Y323A , ptsN H66A spoT Y323A , ptsN H66E spoT Y323A and Δ ptsP spoT Y323A with (dark grey bars) or without (light grey bars) P xylX::relA-FLAG in PYE medium supplemented with 0.1% of xylose. The data were normalized to the WT without P xylX::relA-FLAG (100%). Error bars=s.d. ; n =3. ( d ) The hydrolase activity of SpoT is required to degrade (p)ppGpp in +N condition. Intracellular levels of (p)ppGpp detected by TLC after nucleotides extraction of spoT Y323A , spoT D81G Y323A , ptsN H66A spoT Y323A and Δ ptsP spoT Y323A containing P xylX::relA-FLAG in +N or −N medium supplemented with 0.1% xylose. Full size image Adaptation to starvation conditions requires sophisticated regulatory mechanisms that sense an external stimulus and translate it into an internal molecular response. In this report, we uncovered how Caulobacter copes with nitrogen starvation by triggering (p)ppGpp accumulation ( Fig. 8 ), which in turn will control the cell cycle and development by extending the G1/swarmer phase [14] , [16] . Increasing the time spent in the non-replicative (G1), motile phase reflects the adaptation of Caulobacter cells to their natural environment, that is, freshwater in which nutrients can rapidly be limiting [3] , [4] . Interestingly, G1 arrest also occurs during the intracellular trafficking of Brucella abortus , and on nitrogen and carbon starvation in Sinorhizobium meliloti [25] , [26] . In addition, the G1 block encountered by S. meliloti cells starved for nitrogen and carbon is also dependent on (p)ppGpp [26] , [27] . Therefore, (p)ppGpp-dependent mechanisms delaying DNA replication initiation could be a common feature used by α-proteobacteria in response to harsh conditions such as infection or starvation. As previously suggested in the literature [5] , our data indicate that stalked cells are able to complete replication upon nitrogen starvation, supporting that only swarmer cells are responsive to nitrogen depletion. Indeed, even if the speed of chromosome duplication is slowed down in nitrogen-starved conditions, the stalked cell seems to be unable to stop ongoing DNA replication ( Supplementary Fig. 1f ). In contrast, the swarmer cell can avoid DNA replication initiation in the same conditions ( Supplementary Fig. 1a–e ). One reason for this difference could be that initiating DNA replication without enough nitrogen supplies would ultimately be detrimental to the cells. In support of this, we showed that deletion of spoT is deleterious in a Δ glnD background, since Δ glnD Δ spoT strain displays a strong growth defect ( Fig. 3b ). This result highlights the importance for Caulobacter swarmer cells to delay DNA replication until reaching a critical intracellular nitrogen pool. Our data established that glutamine deprivation constitutes the intracellular signal perceived by the cell in response to nitrogen starvation and is sufficient to mediate (p)ppGpp accumulation ( Fig. 8 ). Intracellular glutamine concentration is known to vary in bacteria, up to 10-fold depending on nitrogen availability [28] . As a consequence, monitoring intracellular glutamine concentration is an efficient strategy to evaluate nitrogen availability, and subsequently adjust nitrogen assimilation. In E. coli , the uridylyltransferase GlnD is known to directly sense the intracellular glutamine pool, and according to it, to modify uridylylation level of regulatory PII proteins (GlnB and GlnK), which in turn will adapt nitrogen metabolism. For instance, in the absence of glutamine, GlnD will increase ammonium transport, as well as the expression and activity of the glutamine synthetase. Intriguingly, three GlnA paralogs are encoded into the genome of C. crescentus , suggesting a functional redundancy, and the presence of multiple glutamine synthetase is conserved in several α-Proteobacteria [29] . Even though we showed that only the glutamine synthetase encoded by glnA is necessary for assimilating ammonium in complex and minimal media, we do not exclude that the two other paralogs (GlnA 2 and GlnA 3 ) display a glutamine synthetase activity under specific growth conditions that remain to be determined. Glutamine synthetase activity has been shown to promote growth of the obligatory intracellular α-proteobacterium Ehrlichia chaffeensis inside human cells [30] . Moreover, this successful intracellular growth of E. chaffeensis promoted by the glutamine pool was accompanied by a rapid degradation of CtrA, a cell cycle regulator known to inhibit DNA replication initiation in several α-proteobacteria [7] , [31] . Furthermore, the CtrA level in Caulobacter cells was shown to be maintained upon nitrogen starvation [5] , and even increased upon (p)ppGpp accumulation [16] . These observations suggest that the asymmetrically dividing α-proteobacteria might use glutamine as a metabolic cue for nitrogen availability that controls the cell cycle thanks to (p)ppGpp alarmone. It would be interesting to check if the PTS Ntr system is used by other α-proteobacteria to relay nitrogen starvation (glutamine deprivation) to (p)ppGpp production and subsequent G1 arrest. Only a few mechanisms triggering (p)ppGpp accumulation in nutrient-limiting conditions have so far been deciphered at the molecular level [8] . When E. coli cells are starved for amino acids, the (p)ppGpp synthetase RelA is directly activated by ribosomes whose A site is occupied by an uncharged tRNA [32] , whereas the bifunctional (p)ppGpp synthetase/hydrolase SpoT is regulated by an acyl carrier protein in response to fatty acid starvation [33] , [34] . In this report, we discovered a new molecular mechanism stimulating (p)ppGpp accumulation in response to nutrient starvation. This mechanism involves the PTS Ntr system as an important metabolic sensor that translates a glutamine deprivation signal into a (p)ppGpp accumulation signal. Our data suggest that EIIA Ntr ∼ P directly reduces the hydrolase activity of SpoT, while HPr ∼ P indirectly activates (p)ppGpp production upon nitrogen starvation ( Fig. 8 ). Historically, the PTS system was discovered as a phosphorylation cascade involved in the regulation of sugar uptake and carbon catabolite repression [21] , [35] . Afterwards, a second phosphotransferase system (PTS Ntr ) was proposed to be connected to nitrogen metabolism but this connection remained poorly described [21] . The direct inhibition of EI Ntr autophosphorylation by glutamine observed in E. coli and S. meliloti [22] , [36] , as well as now in C. crescentus ( Fig. 4 ), reinforces the idea that nitrogen constitutes a signal for PTS Ntr systems. The fact that the GAF domain, highly conserved in all EI Ntr proteins ( Supplementary Fig. 4b ), is required for binding glutamine suggests that the glutamine-dependent control of EI Ntr phosphorylation might be a common feature in PTS Ntr system. In contrast to its EIIA paralog, the EIIA Ntr component is not associated with permeases, but rather carries out regulatory functions, by interacting with its target(s). For example, the unphosphorylated form of EIIA Ntr inhibits pyruvate dehydrogenase activity in Pseudomonas putida by interacting with the E1 subunit [37] . Our work constitutes so far the first example of regulatory functions mediated by the phosphorylated form of EIIA Ntr (EIIA Ntr ∼ P). Indeed, our results support the conclusion that only the phosphorylated form of EIIA Ntr interacts with SpoT to inhibit its hydrolase activity. This is further supported by the fact that EI Ntr and SpoT are found in the same protein complex during stationary phase [38] . Interestingly, a direct interaction between the non-phosphorylated form of EIIA Ntr and SpoT has been recently found in the β-proteobacterium Ralstonia eutropha by BTH but no function was assigned for this connection [39] . This differential interaction between phosphorylated or non-phosphorylated form EIIA Ntr and SpoT illustrates the evolutionary plasticity of PTS Ntr components with their targets. Besides EIIA Ntr ∼ P, we know that phosphorylated HPr also controls (p)ppGpp accumulation on nitrogen starvation, but how this regulation works at the molecular level remains an open question. HPr ∼ P could interact with an unknown factor (X in Fig. 8 ), which in turn could modulate the abundance of SpoT or activate its synthetase activity, to subsequently increase the global (p)ppGpp pool. Although we have now uncovered the pathway that stimulates (p)ppGpp accumulation in response to nitrogen starvation, understanding how (p)ppGpp affects the G1-to-S transition at the molecular level will be a challenge for future work. Bacterial strains and growth conditions Oligonucleotides, strains and plasmids used in this study are listed in Supplementary Tables 1, 2 and 3 , altogether with construction details provided in the Supplementary Methods . E. coli Top10 was used for cloning purpose, and grown aerobically in Luria–Bertani (LB) broth (Sigma) [40] . Electrocompetent cells were used for transformation of E. coli. All Caulobacter crescentus strains used in this study are derived from the synchronizable wild-type strain NA1000, and were grown in PYE or synthetic M2 (20 mM PO 4 3− , 9.3 mM NH 4 + ; +N) or P2 (20 mM PO 4 3− ; −N) supplemented with 0.5 mM MgSO 4 , 0.5 mM CaCl 2 , 0.01 mM FeSO 4 and 0.2% glucose (M2G or P2G, respectively) media at 28–30 °C. Glutamine (Q) was used at a final concentration of 9.3 mM. Growth was monitored by following the OD (600 nm) during 24 h, in an automated plate reader (Bioscreen C, Lab Systems) with continuous shaking at 30 °C. Genes expressed from the inducible vanA promoter (P vanA ) was induced with 0.5 mM vanillate. Generalized transduction was performed with phage ФCr30 according to the procedure described in ref. 41 . Motility was monitored on PYE swarm (0.3% agar) plates. Area of the swarm colonies were quantified with ImageJ software as described previously in ref. 42 . Motility screen was performed on PYE swarm (0.3% agar) plates supplemented with glutamine (9.3 mM) during 3–4 days at 30 °C. Genomic DNA of the candidates was then sequenced by the Illumina sequencing method (Beckman Coulter Genomics). Transpositional screen was performed with himar1 transposons on PYE plates as previously described in ref. 43 . The exact positions of three himar1 insertion sites into the ptsP locus ( Fig. 3a ) have been determined by semi-arbitrary PCR. The presence of himar1 transposons into the ptsP locus was checked by PCR with primers (926 and 927) hybridizing upstream and downstream of ptsP . For E. coli , antibiotics were used at the following concentrations (μg ml −1 ; in liquid/solid medium): ampicillin (50/100), kanamycin (30/50), oxytetracycline (12.5/12.5). For C. crescentus , media were supplemented with kanamycin (5/20), oxytetracycline (1/2.5) where appropriate. The doubling time of Caulobacter strains was calculated in exponential phase (OD 660 : 0.2–0.5) using D=(ln(2)·(T (B) −T (A) ))/(ln(OD 660(B) )−ln(OD 660(A) )) and normalized according to the wild-type strain. E. coli S17–1 and E. coli MT607 helper strains were used for transferring plasmids to C. crescentus by bi- and tri-parental mating, respectively. In-frame deletions were created by using pNPTS138-derivative plasmids and by following the procedure described previously in ref. 44 . Flow cytometry analysis DNA content was measured using fluorescence-activated cell sorting (FACS). Cells were fixed in ice-cold 70% ethanol. Fixed samples were then washed twice in FACS staining buffer (10 mM Tris pH 7.2, 1 mM EDTA, 50 mM NaCitrate, 0.01% Triton X-100) containing 0.1 mg ml −1 RNaseA and incubated at room temperature (RT) for 30 min. Cells were then collected by centrifugation for 2 min at 8,000 g , resuspended in 1 ml FACS staining buffer containing 0.5 μM Sytox Green Nucleic acid stain (Life Technologies), and incubated at RT in the dark for 5 min. Samples were analysed in flow cytometer (FACS Calibur, BD Biosciences) at laser excitation of 488 nm. At least 1 × 10 4 cells were recorded in triplicate for each experiment. Gate for cells in G1 phase was determined with a sample of wild-type cells treated with Rifampicin (2.5 μg ml −1 ) for 3 h. Percentage of gated G1 cells of each strain was then normalized using gated G1 cells of the wild-type strain as reference. Synchronization of cells For synchrony, cells were grown in 200 ml of PYE (OD 660 ∼ 0.8), collected by centrifugation for 15 min at 6,000 g , 4 °C; resuspended in 60 ml of ice-cold 20 mM phosphate (PO 4 3− ) buffer and combined with 30 ml of Ludox LS Colloidal Silica (30%; Sigma-Aldrich) [45] . Cells resuspended in Ludox was centrifuged for 40 min at 9,000 g , 4 °C. Swarmer cells, corresponding to the bottom band, were isolated, washed twice in ice-cold PO 4 3− buffer and finally resuspended in prewarmed PYE media for growth at 30 °C. Samples were collected every 15 min for western blot, microscopy and FACS analyses. Light and fluorescent microscopy All strains were imaged during exponential growth phase after immobilization on 1% agarose pads [41] . Microscopy was performed using Axioskop microscope (Zeiss), Orca-Flash 4.0 camera (Hamamatsu) and Zen 2012 software (Zeiss). Images were processed with ImageJ. Supplementary Movie 1 was done with Debut Video Capture Software. Detection of intracellular (p)ppGpp levels (p)ppGpp levels were visualized as described previously in ref. 13 . Briefly, strains were grown overnight in PYE and then diluted for a second overnight culture in M5GG (low-phosphate medium M5G supplemented with 1 mM glutamate). Then, cells were diluted a second time in M5GG and grown for 3 h to reach an OD 660 of 0.4. Cells were split into two parts and washed twice with P5G-labelling buffer (M5G without NH 4 + and with 12.2 mM NaCl and 3.9 mM KCl instead of Na 2 HPO 4 and KH 2 PO 4 ). In all, 1 ml of cells were then resuspended in 225 μl of P5G-labelling (−N) or M5G-labelling (+N) supplemented with 25 μl of KH 2 32 PO 4 at 100 μCi ml −1 and incubated for 2 h with shaking (450 r.p.m.) at 30 °C. Then, samples were extracted with an equal volume of 2 M formic acid, placed on ice for 30 min and then stored overnight at −20 °C. All cell extracts were pelleted at 18,000 g for 3 min and 6 × 2 μl of supernatant was spotted onto a polyethyleneimine plate (Macherey-Nagel). Polyethyleneimine plates were then developed in 1.5 M KH 2 PO 4 (pH 3.4) at RT. Finally, TLC plates were imaged on a MS Storage Phosphor Screen (GE Healthcare) and analysed with Cyclone Phosphor Imager (PerkinElmer). For hydrolase experiments ( Fig. 7d ), cells were incubated 1 h in P5G supplemented with xylose (0.1%). Then, cells were washed twice with P5G-labelling and resuspended in P5G-labelling (−N) supplemented with KH 2 32 PO 4 , xylose (0.1%) and with (+N) or without (−N) glutamine (9.3 mM). BTH assays BTH assays were performed as described previously in refs 23 and 42 . Briefly, 2 μl of MG1655 cyaA::frt (RH785), MG1655 cyaA::frt Δ npr (RH2122), MG1655 cyaA::frt Δ ptsP Δ ptsI (RH2124) strains expressing T18 and T25 fusions were spotted on MacConkey Agar Base plates supplemented with ampicillin, kanamycin, maltose (1%) and IPTG (1 mM) and incubed for 3–4 days at 30 °C. All proteins were fused to T25 at their N-terminal extremity (pKT25) or to the T18 at their N- (pUT18C) or C-terminal (pUT18) extremity. BTH assays in both directions (T25-X with T18-Y or T25-Y with T18-X) gave similar results. The β-galactosidase assays were performed as described in ref. 46 . Briefly, 50 μl E. coli BTH strains cultivated overnight at 30 °C in LB medium supplemented with kanamycin, ampicillin and IPTG (1 mM) were resuspended in 800 μl of Z buffer (60 mM Na 2 HPO 4 , 40 mM NaH 2 PO 4 , 10 mM KCl, 1 mM MgSO 4 ) and lysed with chloroform. After the addition of 200 μl ONPG (4 mg ml −1 ), reactions were incubated at 30 °C until colour turned yellowish. Reactions were then stopped by the addition of 500 μl of 1 M Na 2 CO 3 , and absorbance at 420 nm was measured. Miller units are defined as (OD 420 × 1,000)/(OD 590 × t × v), where, ‘OD 590 ’ is the absorbance at 590 nm of the cultures before the β-galactosidase assays, ‘t’ is the time of the reaction (min) and ‘v’ is the volume of cultures used in the assays (ml). All the experiments were performed with three biological replicates and Miller units of the T25-X T18-ZIP combination were used as a blank and substracted. Immunoblot analysis Immunoblot analyses were performed as described in ref. 46 , with the following primary antibodies: α-Flagellin (1:5,000; ref. 47 ), α-FLAG (1:5,000; Stratagene), α-MreB (1:5,000; ref. 46 ) and secondary antibodies: 1:10,000 anti-mouse (for α-FLAG) or 1:7,500 anti-rabbit (for all the others) linked to peroxidase (GE Healthcare), and visualized thanks to Western Lightning Plus-ECL chemiluminescence reagent (Biorad) and ImageQuant LAS400 (GE Healthcare). Preparation of fractions containing EI Ntr or EI Ntr L83Q Fractions containing EI Ntr or EI Ntr L83Q proteins were purified from NA1000 and NA1000 ptsP L83Q (RH1748) strains, respectively. C. crescentus strains were grown in 150 ml PYE liquid media (OD 660 ∼ 0.7), collected by centrifugation for 15 min at 6,000 g , 4 °C, washed by ice-cold 20 mM phosphate buffer and then resuspended in 5 ml ice-cold phosphate buffered-saline containing 0.05% Triton X-100, complete EDTA-free anti-proteases, 20 mg ml −1 lysozyme, 10 U ml −1 DNase I. Cells were first lysed by sonication, then zirconium beads were added and cells were disrupted by Fastprep cycles (5 × 20 s). Lysates were pelleted at 15 000g at 4 °C and then resuspended in 500 μl of buffer containing 25 mM Tris/HCl pH 7.5, 10 mM MgCl 2 , 1 mM DTT. Autophosphorylation levels of EI Ntr and EI Ntr L83Q [ 32 P]PEP was prepared enzymatically as described previously in ref. 48 . Briefly, 50 μl reaction solution containing 100 mM triethylamine/HCl pH 7.6, 15 mM KCl, 3 mM MgCl 2 , 165 μM PEP, 1 mM pyruvate, 5 μM ATP, 60 μCi [γ- 32 P]-ATP (5,000 Ci mmol −1 ) and 40 units of pyruvate kinase (Sigma) were incubated at 30 °C for 2 h. Phosphorylation assays were performed in 20 μl of solution containing 10 μl of proteins extract (containing EI Ntr or EI Ntr L83Q ), 25 mM Tris/HCl pH 7.5, 10 mM MgCl 2 , 1 mM DTT, glutamine (0, 2, 5 or 10 mM) and 0.5 μl of [ 32 P]PEP solution at 37 °C for 30 min. Then, 5 μl of 5 × SDS-PAGE loading buffer were added to the samples. Proteins were subjected to electrophoresis in a 10% SDS-polyacrylamide gel. SDS-polyacrylamide gels were then dried and imaged on a MP Phosphor system (Packard) and analysed with Cyclone Phosphor Imager (PerkinElmer). Analysis of radioactive spots reveals three bands at different size ( ∼ 50, 80 and 90 kDa). The band corresponding to ∼ 80 kDa, absent in protein extracts from the Δ ptsP strain, was determined as EI Ntr or EI Ntr L83Q . In vivo phosphorylation of EIIA Ntr Strains containing pXMCS2 -3FLAG-ptsN were grown overnight in PYE supplemented with kanamycin and then diluted for a second overnight culture in M5GG (low-phosphate medium M5G supplemented with 1 mM glutamate) supplemented with kanamycin. Then, cells were diluted in M5GG with or without xylose (0.1%), and grown for 3 h to reach an OD 660 of 0.5. In all, 1 ml of cells were washed twice with P5G-labelling buffer (M5G without NH 4 + and with 12.2 mM NaCl and 3.9 mM KCl instead of Na 2 HPO 4 and KH 2 PO 4 ). Cells were then resuspended in 225 μl of P5G-labelling, P5X-labelling (xylose 0.1%) or P5XQ-labelling (xylose 0.1%, glutamine 9.3 mM) supplemented with 25 μl of KH 2 32 PO 4 at 100 μCi ml −1 and incubated for 2 h with shaking (450 r.p.m.) at 30 °C. Samples were collected for 2 min at 12,000 r.p.m., resuspended in 50 μl of lysis buffer (50 mM Tris pH 7.0, 80 mM EDTA, 150 mM NaCl, 4% Triton X-100) and incubated for 2 min at 4 °C. Then, 900 μl of low-salt buffer (50 mM Tris pH 7.0, 100 mM NaCl, 50 mM EDTA, 2% Triton X-100) were added and samples were collected for 15 min at 4 °C. Supernatants were mixed with anti-FLAG M2 magnetic beads (Sigma) previously washed three times with TBS buffer and twice with low-salt buffer. Samples were incubated on a rotating shaker for 90 min at 4 °C, and beads were washed once with cold low-salt buffer and twice with cold high-salt buffer (50 mM Tris pH 7.0, 500 mM NaCl, 50 mM EDTA, 0.1% Triton X-100). Magnetic beads were then resuspended in 20 μl of 3 × SDS loading buffer and 5 μl of 0.5 mg ml −1 of 3FLAG peptide (Sigma) were added to each sample. After 10 min incubation with shaking (1,300 r.p.m. ), proteins were subjected to electrophoresis in a 12% SDS-polyacrylamide gel. SDS-polyacrylamide gels were then dried and imaged on a MP Phosphor system (Packard) and analysed with Cyclone Phosphor Imager (PerkinElmer). Band intensities were quantified with ImageJ software by using the WT (−Xyl, −N) as the background. How to cite this article: Ronneau, S. et al . Phosphotransferase-dependent accumulation of (p)ppGpp in response to glutamine deprivation in Caulobacter crescentus . Nat. Commun. 7:11423 doi: 10.1038/ncomms11423 (2016).